MtDNA mutagenesis impairs elimination of mitochondria during erythroid maturation leading to enhanced erythrocyte destruction Haematopoietic progenitor cells show special sensitivity to mitochondrial DNA (mtDNA) mutagenesis, which suggests that increased mtDNA mutagenesis could underlie anemias. Here we show that elevated mtDNA mutagenesis in mice with a proof-reading deficient mtDNA polymerase ( PolG ) leads to incomplete mitochondrial clearance, with asynchronized iron loading in erythroid precursors, and increased total and free cellular iron content. The resulting Fenton chemistry leads to oxidative damage and premature destruction of erythrocytes by splenic macrophages. Our data indicate that mitochondria actively contribute to their own elimination in reticulocytes and modulate iron loading. Asynchrony of this sequence of events causes severe mitochondrial anaemia by depleting the organism of red blood cells and the bone marrow of iron. Our findings account for the anaemia development in a progeroid mouse model and may have direct relevance to the anemias associated with human mitochondrial disease and ageing. Mitochondrial dysfunction leads to a plethora of human diseases with variable manifestations and age of onset, with anaemia being a severe manifestation in a subset of these disorders [1] , [2] . Pearson’s syndrome is a sporadic infant-onset mitochondrial disorder caused by a heteroplasmic mitochondrial DNA (mtDNA) deletion and characterized by severe anaemia. This multi-organ disorder is often fatal during early years of life [3] , [4] . These patients have been reported to have vacuolization of bone-marrow precursors [4] , but the pathogenic mechanisms of Pearson’s anaemia are unknown. Some patients recover from the blood manifestation after the first years of life along with the loss of mtDNA deletion in leucocytes [4] . Similar to patients with Pearson’s syndrome, mice carrying a heteroplasmic primary single mtDNA deletion (Mitomice) develop anaemia and kidney dysfunction, and die at 6 months of age [5] , [6] . Anaemia is also a manifestation of the progeroid mtDNA mouse model known as the ‘Mutator’, which harbours a proof-reading deficient mtDNA polymerase gamma ( PolG ) that leads to increased random mtDNA mutagenesis in all cell types, including somatic stem cells (SSCs) [7] , [8] , [9] . These mice show aberrant hematopoiesis that initiates in embryogenesis and is progressive, developing anaemia and leucopenia after 6 months of age ultimately restricting their lifespan to about 50 weeks of age [9] . However, even on terminal-stage anaemia the Mutator bone marrow contains all the different erythroid progenitor populations and the total cellularity is not decreased [9] , [10] . Therefore, exhaustion of the haematopoietic stem cell (HSC) pool does not account for the severe anaemia of these mice. The Mitomice and Mutators are the only mouse models with constitutive mitochondrial dysfunction that manifest with anaemia. Why the haematopoietic compartment is spared in other human mitochondrial disorders and mouse models is currently unknown. Several hypotheses could account for the effect: (1) the causative mtDNA mutation is selected against in proliferating cells, as occurs in Pearson syndrome patients that survive the anaemia; (2) mtDNA mutagenesis is slowly progressive and/or does not affect the erythroid cells (adult-onset mtDNA maintenance disorders) (3) the specific mitochondrial pathway is redundant [11] , [12] . For example, Deletor mice [12] carry a mutation in the nuclear-encoded replicative Twinkle helicase, leading to subtle progressive accumulation of secondary multiple mtDNA deletions after 1 year of age. These mice only show mtDNA mutagenesis in postmitotic tissues, not in SSCs, and accordingly do not develop anaemia [9] . Mitochondria are required for haeme biosynthesis and thus critical in the key maturation steps of the erythroid lineage. When the haemoglobin synthesis reaches a threshold the erythrocyte precursors enucleate, and the immature erythrocytes—the reticulocytes—exit the bone marrow and enter the blood circulation. The final maturation of the erythrocytes, including clearance of the remaining organelles and the transferrin receptor (TfR), occurs in the peripheral blood. Mitochondrial removal from maturing erythrocytes occurs by degradation [13] , [14] , [15] the signalling of which is only starting to be unravelled. Mitophagy in erythroid maturation depends on Atg7 or Unc-51-like kinase 1 (Ulk1)-dependent pathways [15] , [16] , [17] with the latter suggested to be most important for mitophagy in foetal definitive reticulocytes [18] . BCL2-related protein NIX (BNIP3L) has been shown to mark mitochondria for mitophagy [19] , [20] , and to be important for the known macroautophagic mechanisms of mitochondrial clearance. The active destruction of mitochondria renders the mature red blood cells completely devoid of the organelles. Removal of oxygen metabolizing mitochondria from iron-loaded erythrocytes is essential to prevent oxidative damage in mature erythrocytes. Typically in biological systems iron is protein bound [21] , in a reduced state, which is required for haeme biosynthesis and oxygen binding [22] . However, in pathological conditions, such as those inducing superoxide production from the mitochondrial respiratory chain (RC), iron can be released from protein complexes or cofactors, including haeme [23] . Free iron is highly reactive with oxygen, and leads to a vicious circle of reactive oxygen species (ROS) generation by Fenton reaction. The free redox-active, non-protein-bound iron (NPBI) further promotes oxidative stress by oxidating, for example, polyunsaturated fatty acids of the membranes, creating reactive aldehydes, including 4-hydroxy-2-nonenal (4-HNE) [23] , [24] . 4-HNE forms stable adducts with amino acid residues cysteine, histidine and lysine, thereby modifying protein function [25] . Moreover, in erythrocytes, oxidative damage can impair flippase activity required to sequester phospholipid phosphatidylserine (PS) to the inner monolayer of the cell membrane [26] , [27] . Exposure of PS on the erythrocyte surfaces acts as a signal for splenic macrophages to capture and destroy old erythrocytes [28] thereby contributing to anaemia. In addition to the damaging effects of oxidative stress, ROS, especially H 2 O 2 , are an important source of signalling molecules for HSC fate determination and differentiation [29] , [30] , [31] , [32] . In Mutators, the redox-active antioxidant N -Acetyl- L -cysteine (NAC) rescued the erythroid and lymphoid differentiation in embryonal haematopoiesis, indicating that subtle increases in ROS signalling by mtDNA mutagenesis disturbed SSC homoeostasis [9] . We show that elevated mtDNA mutagenesis impairs erythrocyte maturation by delaying mitochondrial and TfR clearance, increasing free iron, erythrocyte lipid oxidation and membrane modification, which altogether shortens the lifespan of the erythrocytes because of their accelerated destruction in the spleen. Our results suggest that mitochondria have an active role in their own removal from maturing erythrocytes, and based on these findings we propose a novel mechanism for mitochondrial anaemia. Mutator blood contains erythrocytes carrying mitochondria At 11 months of age, Mutator mice developed terminal anaemia, with blood haemoglobin content as low as 50 g l −1 , with a significant proportion of bone-marrow erythroid precursors showing an abnormal precursor identity [9] , [10] . At this age, the Mutators showed increased reticulocyte amounts in their peripheral blood, a feature consistent with severe anaemia (Mutator 7.4±2.6% of total erythrocytes, n =11; wild type (WT) 3.3±0.6%, n =11; P <0.0001, Student’s t -test). However, these reticulocytes were immature ( Fig. 1a ) and had fourfold increased content of TfR and eightfold increased content of mitochondria ( Fig. 1b,c ). 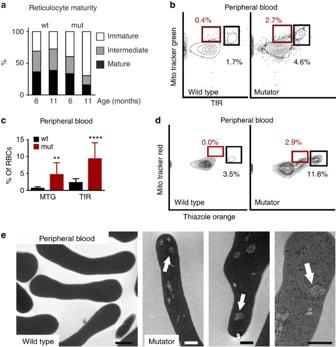Figure 1: Erythrocytes carry mitochondria in mitochondrial DNA mutator mouse. (a) Reticulocyte maturity staged by ribosomal RNA content (thiazole orange) in the peripheral blood at the age of 11 months. Mutator (mut) mice showed an increased proportion of immature reticulocytes (two-tailedP<0.0001, Student’st-test). Age 6 months: WTn=5, Mutatorn=4; age 11 months: WTn=11, Mutatorn=11 (30,000 cells per sample were analyzed). (b) Representative FACS plot and (c) quantification of transferrin receptor (TfR) amount and mitochondria (MitoTracker Green) in Mutator erythrocytes at the age of 11 months (two-tailedP<0.0001 andP=0.0059, respectively, Student’st-test). WT:n=12, Mutator:n=8 (30,000 cells per sample were analyzed). Data are presented as mean±s.d. (d) A representative FACS plot of ribosomes (thiazole orange, TO) and mitochondria (MitoTracker Red); black box: reticulocytes positive for both TO and MTR; red box: abnormal population carrying mitochondria. (e) Electron micrograph of peripheral blood erythrocytes at 8 months of age. WT erythrocytes: biconcave morphology, no organelles; Mutator erythrocytes (three separate figures) contained mitochondria (arrows). WT scale bar, 1 μm, Mutator scale bar, 0.5 μm. See alsoSupplementary Fig. 1. Figure 1: Erythrocytes carry mitochondria in mitochondrial DNA mutator mouse. ( a ) Reticulocyte maturity staged by ribosomal RNA content (thiazole orange) in the peripheral blood at the age of 11 months. Mutator (mut) mice showed an increased proportion of immature reticulocytes (two-tailed P <0.0001, Student’s t -test). Age 6 months: WT n =5, Mutator n =4; age 11 months: WT n =11, Mutator n =11 (30,000 cells per sample were analyzed). ( b ) Representative FACS plot and ( c ) quantification of transferrin receptor (TfR) amount and mitochondria (MitoTracker Green) in Mutator erythrocytes at the age of 11 months (two-tailed P <0.0001 and P =0.0059, respectively, Student’s t -test). WT: n =12, Mutator: n =8 (30,000 cells per sample were analyzed). Data are presented as mean±s.d. ( d ) A representative FACS plot of ribosomes (thiazole orange, TO) and mitochondria (MitoTracker Red); black box: reticulocytes positive for both TO and MTR; red box: abnormal population carrying mitochondria. ( e ) Electron micrograph of peripheral blood erythrocytes at 8 months of age. WT erythrocytes: biconcave morphology, no organelles; Mutator erythrocytes (three separate figures) contained mitochondria (arrows). WT scale bar, 1 μm, Mutator scale bar, 0.5 μm. See also Supplementary Fig. 1 . Full size image The flow cytometric analysis showed that a subset of mature erythrocytes of the Mutator mice had no or few ribosomes, but contained mitochondria ( Fig. 1d red box), which was further verified by electron microscopy of the Mutator peripheral blood ( Fig. 1e ). This was never observed in the WT mice. In the biconcave erythrocytes carrying mitochondria, 9% of the organelles were surrounded by autophagic membranes ( Supplementary Fig. 1 ). This suggested that mitophagy per se was slowed down in the Mutators or that a decreased number of mitochondria were marked for clearance. We also observed in the electron microscopic analysis of the Mutator erythrocytes the presence of electron-dense cytoplasmic speckles, more dense than ribosomes, reminiscent of metal accumulation. These features were not observed in WT mature biconcave erythrocytes. Together these data suggest that elevated mtDNA mutagenesis severely disturbs mitochondrial degradation during erythroid maturation. Mutator reticulocytes have delayed mitochondrial clearance To study in detail the impact of mtDNA mutagenesis on erythroid maturation, we established in vitro analysis of Mutator bone-marrow HSCs on methylcellulose. This indicated that their erythroid differentiation was significantly delayed, but not completely stalled ( Fig. 2a ). The typical reddish, haemoglobin-containing erythroid progenitor colonies were apparent in Mutator samples only after 12 days of culture, whereas WT HSCs formed colonies already in a week ( Fig. 2b ). We then established reticulocyte culture to investigate the dynamics of erythroid maturation, especially focusing on mitochondrial degradation. We stimulated reticulocytosis by serial phlebotomy in young, pre-anaemic Mutators, and cultured the reticulocytes in vitro . Both Mutator and WT mice produced large amounts of reticulocytes (Mutator: 13.8±1.1%, n =5; WT: 14.7±0.7%, n =5), indicating similar capacity of their bone marrow for stress-induced erythropoiesis. However, the Mutator reticulocytes showed significantly delayed mitochondrial removal ( Fig. 2c ), whereas ribosomal RNA clearance was similar to WT ( Supplementary Fig. 2a ). Three days post harvest, only 4.3±0.6% of WT erythroid cells contained mitochondria, whereas 9.3±1.4% of the Mutators still had mitochondria ( P =0.0003, Student’s t -test) ( Fig. 2d ). Ultrastructural analysis of the blood after the serial phlebotomy confirmed in the Mutators the presence of morphologically mature biconcave erythrocytes containing mitochondria, while in the WT the only mitochondria-containing cells were round in shape, a feature typical for early reticulocytes ( Supplementary Fig. 2b ). The WT reticulocyte mitochondria lost their membrane potential rapidly in culture followed by organelle disappearance, but Mutators retained mitochondria with membrane potential significantly longer (2 days of culture: WT: 7.9±0.6%, n =4; Mutator: 13.4±2.2%, n =5, P =0.01, Student’s t -test) ( Fig. 2e ). Lysosomes, involved in autophagic clearance, were similar in number in Mutator reticulocytes compared with WT cells (LysoTracker Red® positive cells: WT 2.7±1.4%, Mutator 2.2±0.7%), whereas the protein level of NIX was reduced ( Supplementary Fig. 2c ). These results indicate that mtDNA mutagenesis affects erythrocyte maturation by delaying mitochondrial exclusion in reticulocytes, and that mitochondrial signalling contributes to their own exclusion. 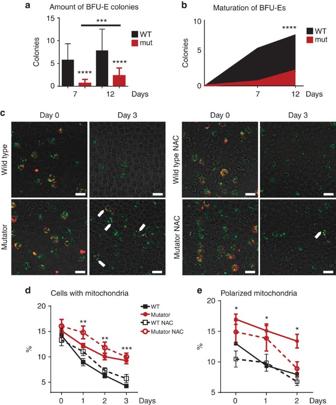Figure 2: Delayed erythroid maturation and mitochondrial clearancein vitro. (a) Colony forming assay for bone-marrow hematopoietic stem cells (Mutator:n=8, WT:n=8, each sample analyzed in triplicate). Mutators showed decreased amount of BFU-E (burst-forming unit, erythroid) colonies (two-tailedP<0.0001, Student’st-test, data are presented as mean±s.d.). (b) Time required to form haemoglobin-containing mature BFU-Es was delayed by 5 days in Mutators compared with WT (P<0.0001, linear regression analysis). (c) Confocal microscopy of cultured reticulocytes from phlebotomized animals with or without NAC treatment: polarized (TMRM in red) and depolarized (MitoTracker Green) mitochondria. Mutator reticulocytes retained mitochondria longer than WT cells; part of the mitochondria were still polarized after 3 days of culture (arrowheads). Scale bars, 10 μm. (d) Quantification of cells with mitochondria (FACS analysis, MTG per total cell count): Mutator reticulocytes retained mitochondria significantly longer than WT, and NAC had no effect on the clearance (WT versus Mutator day 1P=0.004, day 2P=0.002 and day 3P=0.0003, Student’st-test). (e) Quantification of cells with polarized mitochondria (FACS analysis, TMRM per total cell count): NAC increased depolarization of mitochondria in Mutator reticulocytes (WT versus MutatorP=0.01, Mutator versus Mutator NAC day 2P=0.03). For (d,e) WT:n=4, Mutator:n=5, WT NAC:n=6 and Mutator NAC:n=6 (30,000 cells per sample were analyzed). Data are shown as mean±s.d. Figure 2: Delayed erythroid maturation and mitochondrial clearance in vitro. ( a ) Colony forming assay for bone-marrow hematopoietic stem cells (Mutator: n =8, WT: n =8, each sample analyzed in triplicate). Mutators showed decreased amount of BFU-E (burst-forming unit, erythroid) colonies (two-tailed P <0.0001, Student’s t -test, data are presented as mean±s.d.). ( b ) Time required to form haemoglobin-containing mature BFU-Es was delayed by 5 days in Mutators compared with WT ( P <0.0001, linear regression analysis). ( c ) Confocal microscopy of cultured reticulocytes from phlebotomized animals with or without NAC treatment: polarized (TMRM in red) and depolarized (MitoTracker Green) mitochondria. Mutator reticulocytes retained mitochondria longer than WT cells; part of the mitochondria were still polarized after 3 days of culture (arrowheads). Scale bars, 10 μm. ( d ) Quantification of cells with mitochondria (FACS analysis, MTG per total cell count): Mutator reticulocytes retained mitochondria significantly longer than WT, and NAC had no effect on the clearance (WT versus Mutator day 1 P =0.004, day 2 P =0.002 and day 3 P =0.0003, Student’s t -test). ( e ) Quantification of cells with polarized mitochondria (FACS analysis, TMRM per total cell count): NAC increased depolarization of mitochondria in Mutator reticulocytes (WT versus Mutator P =0.01, Mutator versus Mutator NAC day 2 P =0.03). For ( d , e ) WT: n =4, Mutator: n =5, WT NAC: n =6 and Mutator NAC: n =6 (30,000 cells per sample were analyzed). Data are shown as mean±s.d. Full size image Antioxidant is unable to rescue the mitochondrial clearance Previously, we showed that NAC supplementation rescued erythroid differentiation in Mutator-mouse embryos [9] , and therefore we tested whether NAC could affect the maturation and organellar exclusion in Mutator reticulocytes. We administered NAC to Mutators and WT during phlebotomy and reticulocyte culture, but found no effect on mitochondrial clearance ( Fig. 2d ). NAC significantly accelerated mitochondrial depolarization in Mutator reticulocytes ( Fig. 2e ), but did not affect lysosomal content (LysoTracker positive cells: WT 2.7±1.4%, WT NAC 2.8±0.8%, Mutator 2.2±0.7%, Mutator NAC 2.0±0.7%), or increase the amount of NIX protein ( Supplementary Fig. 2c ). These results indicate that ROS/redox signalling is not mediating the mitochondrial removal defect in Mutators, or at least acutely administered NAC is unable to rescue mitochondrial clearance. Mutators develop anaemia despite long-term NAC treatment To test whether NAC treatment could promote erythrocyte maturation, if administered through development and adult life of Mutators in vivo , we performed a long-term NAC treatment trial: Mutators and WT mice were supplemented with NAC, throughout embryogenesis until 11 months of adult age. In contrast to the NAC rescue of the embryonal HSC defect [9] , NAC had no effect on the adult Mutator erythropoiesis defect ( Supplementary Fig. 2e,f ). A similar amount of peripheral blood erythrocytes with mature morphology contained mitochondria in NAC-treated versus non-treated Mutator animals, and 9% of mitochondria were surrounded by autophagic membranes in both groups ( Supplementary Fig. 1 ). These results indicate that mitochondrial ROS/redox signalling contributes differently to haematopoiesis and erythroid differentiation during embryonal and adult life. Mutators show aberrant iron loading and oxidative stress Flow cytometric analysis showed that in addition to mitochondrial presence, iron loading was potentially abnormal: most of the Mutator reticulocytes that retained mitochondria were also TfR positive ( Fig. 1b,c ). Furthermore, in cultured Mutator reticulocytes, TfR localization was abnormal being dispersed throughout the cell membrane and consistent with extended TfR-mediated iron loading. In contrast, in WT reticulocytes the TfR were clustered for exclusion ( Fig. 3a ). NAC treatment rescued the localization of TfR in Mutator cells to be similar to WT ( Fig. 3a ). Extended presence of TfR within the Mutator reticulocytes suggested abnormal iron loading, and indeed, we found the total iron content of Mutator serum as well as transferrin saturation to be significantly increased ( Fig. 3b,c ). Furthermore, free NPBI was increased over twofold in Mutators at the age of 8–10 months, both in erythrocytes ( P <0.001, Student’s t -test) and plasma ( P <0.0001, Student’s t -test) ( Fig. 3d ). Free iron is highly reactive with oxygen, and a potent source of ROS. To test for oxidative stress in erythrocytes, we measured 4-HNE protein adducts as indicators of lipid peroxidation to be 1.7-fold increased in the erythrocyte membranes ( Fig. 3e ) and in plasma (WT: 15±1 a.u., n =6; Mutator: 19±2 a.u. n =8; P =0.0013, Student’s t -test). These results show that mitochondrial exclusion and TfR-mediated iron loading are both affected in Mutator reticulocyte maturation and suggest that mitochondrial ROS/redox signalling guides the timing of transferrin-mediated iron loading. Furthermore, the asynchronized TfR-mediated iron loading results in an increase of free cellular iron and extensive oxidative damage in Mutator erythrocytes. 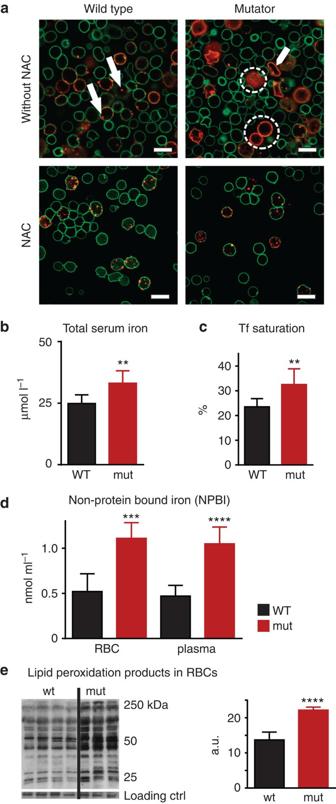Figure 3: Mutator erythrocytes show abnormal iron loading and extensive oxidative damage. (a) Transferrin receptor (red) localization in reticulocytes (Ter119 green) at the second day of culture analyzed by confocal microscopy. WT reticulocytes: most of the TfR was clustered (arrows); Mutator reticulocytes: TfR showed even membrane distribution (dashed circle), even in morphologically mature erythrocytes (arrowhead). NAC treatment rescued TfR distribution in Mutators. WT:n=3, Mutator:n=3, WT NAC:n=3 and Mutator NAC:n=3, samples were analyzed in three separate experiments. Scale bars, 10 μm. (b) Total serum iron level at the age of 10 months (two-tailedP=0.001, Student’st-test). WT:n=6, Mutator:n=17. (c) Transferrin (Tf) saturation at 10 months of age (two-tailedP=0.006, Student’st-test). WT:n=6, Mutator:n=11. (d) Free, non-protein-bound iron (NPBI) in erythrocytes (two-tailedP=0.0002, Student’st-test) and in plasma (two-tailedP<0.0001, Student’st-test) at the age of 8–10 months (WT:n=7, Mutator:n=7, three to five animals were pooled in each sample). (e) 4-hydroxynonenal (4-HNE) protein adducts, lipid peroxidation-induced protein damage, in the erythrocyte membranes at 8–10 months of age (two-tailedP<0.0001, Student’st-test). Representative Western blots shown on left and quantification on right (WT:n=7, mut:n=5, three to five animals were pooled in each sample). Forb–e, data are shown as mean±s.d. Figure 3: Mutator erythrocytes show abnormal iron loading and extensive oxidative damage. ( a ) Transferrin receptor (red) localization in reticulocytes (Ter119 green) at the second day of culture analyzed by confocal microscopy. WT reticulocytes: most of the TfR was clustered (arrows); Mutator reticulocytes: TfR showed even membrane distribution (dashed circle), even in morphologically mature erythrocytes (arrowhead). NAC treatment rescued TfR distribution in Mutators. WT: n =3, Mutator: n =3, WT NAC: n =3 and Mutator NAC: n =3, samples were analyzed in three separate experiments. Scale bars, 10 μm. ( b ) Total serum iron level at the age of 10 months (two-tailed P =0.001, Student’s t -test). WT: n =6, Mutator: n =17. ( c ) Transferrin (Tf) saturation at 10 months of age (two-tailed P =0.006, Student’s t -test). WT: n =6, Mutator: n =11. ( d ) Free, non-protein-bound iron (NPBI) in erythrocytes (two-tailed P =0.0002, Student’s t -test) and in plasma (two-tailed P <0.0001, Student’s t -test) at the age of 8–10 months (WT: n =7, Mutator: n =7, three to five animals were pooled in each sample). ( e ) 4-hydroxynonenal (4-HNE) protein adducts, lipid peroxidation-induced protein damage, in the erythrocyte membranes at 8–10 months of age (two-tailed P <0.0001, Student’s t -test). Representative Western blots shown on left and quantification on right (WT: n =7, mut: n =5, three to five animals were pooled in each sample). For b – e , data are shown as mean±s.d. Full size image Mutator erythrocytes are prematurely captured and destroyed Oxidative damage on erythrocytes is a signal for spleen macrophages to capture the old cells from blood circulation for degradation. Such signal is produced by PS exposure on erythrocyte membrane outer leaflet, resulting from oxidative damage in the enzymes maintaining PS asymmetry. We found that at the age of 8–10 months, Mutator peripheral blood erythrocytes showed a remarkable10-fold increase in PS exposure ( P =0.001, Student’s t -test) ( Fig. 4a and Supplementary Fig. 3a ). The Mutator spleens harboured a 1.9-fold higher amount of erythroid cells than the WT ( P <0.0001, Student’s t -test) ( Fig. 4b ), consistent with extra-medullary haematopoiesis described in these animals [8] , but these cells showed a 5.5-fold increase in PS exposure ( P <0.0001, Student’s t -test) ( Fig. 4c and Supplementary Fig. 3a ), indicating an increased amount of aged erythrocytes in the spleen. Furthermore, the amount of active splenic macrophages (CD45+, mac3+) that capture damaged erythrocytes for destruction, was twofold in Mutators, when compared with WT ( P =0.0001, Student’s t -test) ( Fig. 4d ), and the macrophages were loaded with iron ( Fig. 4e ). These data indicate enhanced splenic destruction of erythrocytes. However, the Mutator bone marrow showed very low iron amount ( Fig. 4f ). These findings suggested premature aging and shortened lifespan of the Mutator erythrocytes. To assess the lifespan directly, we biotin-labelled the circulating erythrocytes of moderately anaemic 6-month-old Mutators, and monitored their clearance for 3 weeks. Indeed, the Mutator erythrocytes showed significantly decreased lifespan compared with WT littermates ( P =0.03, linear regression analysis) ( Fig. 4g ). Furthermore, Mutator peripheral blood and spleen erythrocytes showed increased levels of CD47 ( Supplementary Fig. 3b ), suggesting that the circulating Mutator erythrocytes were newly formed. These results suggest that Mutator erythrocytes aged prematurely and were degraded soon after their release from the bone marrow. The extensive destruction of erythrocytes in the spleen depleted bone marrow of iron, which further exacerbated the anaemia. 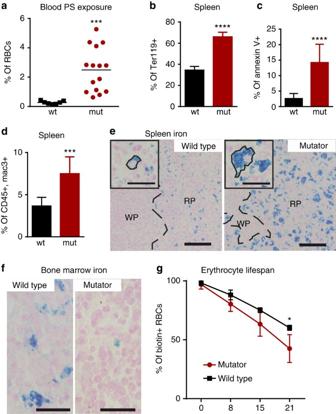Figure 4: Mutator erythrocytes are prematurely destroyed by the spleen macrophages. (a) FACS analysis and quantification of phosphatidylserine (PS) exposure in peripheral blood erythrocytes at the age of 8 months (two-tailedP=0.001, Student’st-test). WT:n=7, Mutator:n=15 (30,000 cells analyzed per sample). (b) FACS analysis and quantification of total amount of erythroid cells (Ter119+) in the spleen (two-tailedP<0.0001, Student’st-test); (c) phosphatidylserine exposure in splenic erythroid cells in Mutator versus WT at the age of 8 months (two-tailedP<0.0001, Student’st-test). WT:n=9, Mutator:n=9 (30,000 cells analyzed per sample). (d) The amount of activated macrophages (CD45+, mac3+) in the spleen at the age of 8 months (two-tailedP=0.0001, Student’st-test). WT:n=9, Mutator:n=9 (30,000 cells analyzed). (e) Histological analysis of iron (blue) in the spleen red pulp (RP, WP=white pulp) at the age of 8 months (WT:n=5, Mutator:n=5, six to nine histological sections were analyzed per sample). Solid line in inset: individual macrophage. Scale bars, 50 μm, inset scale bars, 25 μm. (f) Histological analysis of iron (blue) in the bone marrow at the age of 10 months (WT:n=5, Mutator:n=5, six to nine histological sections were analyzed per sample). Scale bars, 25 μm. (g)In vivoerythrocyte lifespan in 6-month-old Mutators and WT: 30% less Mutator erythrocytes survived 21 days in circulation when compared with WT cells (two-tailedP=0.03, linear regression analysis). WT:n=3, Mutator:n=3 (FACS analysis; 30,000 cells analyzed per sample per timepoint). Forb–d,g, data are shown as mean±s.d. Figure 4: Mutator erythrocytes are prematurely destroyed by the spleen macrophages. ( a ) FACS analysis and quantification of phosphatidylserine (PS) exposure in peripheral blood erythrocytes at the age of 8 months (two-tailed P =0.001, Student’s t -test). WT: n =7, Mutator: n =15 (30,000 cells analyzed per sample). ( b ) FACS analysis and quantification of total amount of erythroid cells (Ter119+) in the spleen (two-tailed P <0.0001, Student’s t -test); ( c ) phosphatidylserine exposure in splenic erythroid cells in Mutator versus WT at the age of 8 months (two-tailed P <0.0001, Student’s t -test). WT: n =9, Mutator: n =9 (30,000 cells analyzed per sample). ( d ) The amount of activated macrophages (CD45+, mac3+) in the spleen at the age of 8 months (two-tailed P =0.0001, Student’s t -test). WT: n =9, Mutator: n =9 (30,000 cells analyzed). ( e ) Histological analysis of iron (blue) in the spleen red pulp (RP, WP=white pulp) at the age of 8 months (WT: n =5, Mutator: n =5, six to nine histological sections were analyzed per sample). Solid line in inset: individual macrophage. Scale bars, 50 μm, inset scale bars, 25 μm. ( f ) Histological analysis of iron (blue) in the bone marrow at the age of 10 months (WT: n =5, Mutator: n =5, six to nine histological sections were analyzed per sample). Scale bars, 25 μm. ( g ) In vivo erythrocyte lifespan in 6-month-old Mutators and WT: 30% less Mutator erythrocytes survived 21 days in circulation when compared with WT cells (two-tailed P =0.03, linear regression analysis). WT: n =3, Mutator: n =3 (FACS analysis; 30,000 cells analyzed per sample per timepoint). For b – d , g , data are shown as mean±s.d. Full size image Human Pearson’s anaemia shares similar maturation defect As mtDNA mutagenesis induced anaemia in mice, we asked the question whether the pathogenesis was similar in human patients with anaemia due to mtDNA mutation. To test this idea, we obtained a rare blood sample from a 22-month old girl suffering from Pearson’s syndrome in acute anaemic state. She showed reticulocytosis, with 4.5-fold increased amount of reticulocytes ( Fig. 5a , dashed boxes), as a compensatory mechanism for anaemia. Similar to the Mutator-mouse model, a subset of mature erythrocytes contained mitochondria, but were devoid of ribosomes ( Fig. 5a , red boxes). Electron microscopic analysis showed that a subset of peripheral erythrocytes possessed an abnormal membrane structure ( Fig. 5b ) and mitochondria. This Pearson’s syndrome patient spontaneously recovered from the anaemia, after which no abnormal cells with organelles were found, either by fluorescence-activated cell sorting (FACS) analysis ( Fig. 5a solid box) or by electron microscopy ( Fig. 5b ). These results suggest that Pearson’s syndrome anaemia is associated with an erythroid maturation defect with delayed mitochondrial clearance, highly similar to the findings we observed in the Mutator-mouse model. 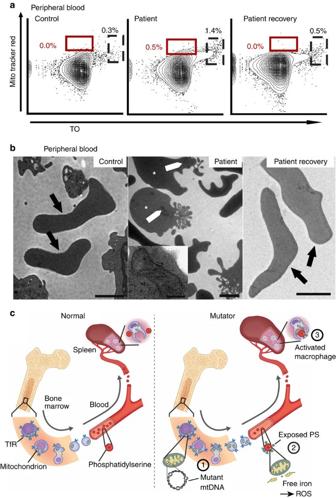Figure 5: Pearson’s patient shows mitochondria in peripheral blood erythrocytes. (a) FACS analysis of peripheral blood. TO: ribosomes; MitoTracker Red: mitochondria. Reticulocytes (dashed box); abnormal cell population with mitochondria (red box). (b) Ultrastructure of peripheral blood erythrocytes of a healthy individual (left), the Pearson’s patient in acute anaemic phase (middle) with morphologically abnormal erythrocytes (asterisk) carrying mitochondria (arrowheads), and Pearson patient after anaemia recovery with only mature erythrocytes similar to control (arrows). Scale bars, 2 μm; inset scale bar, 200 nm. (c) Pathomechanistic model for mitochondrial anaemia. (1) Primary mtDNA mutagenesis induces slow maturation of erythroblasts and delayed mitochondrial clearance from reticulocytes (2) with delayed TfR exclusion, extended iron loading, increase of total iron, increase of free iron, extensive oxidative stress with membrane phosphatidylserine (PS) exposure in the peripheral erythrocytes, which (3) activates splenic macrophages and leads to premature destruction of the erythrocytes. Figure 5: Pearson’s patient shows mitochondria in peripheral blood erythrocytes. ( a ) FACS analysis of peripheral blood. TO: ribosomes; MitoTracker Red: mitochondria. Reticulocytes (dashed box); abnormal cell population with mitochondria (red box). ( b ) Ultrastructure of peripheral blood erythrocytes of a healthy individual (left), the Pearson’s patient in acute anaemic phase (middle) with morphologically abnormal erythrocytes (asterisk) carrying mitochondria (arrowheads), and Pearson patient after anaemia recovery with only mature erythrocytes similar to control (arrows). Scale bars, 2 μm; inset scale bar, 200 nm. ( c ) Pathomechanistic model for mitochondrial anaemia. (1) Primary mtDNA mutagenesis induces slow maturation of erythroblasts and delayed mitochondrial clearance from reticulocytes (2) with delayed TfR exclusion, extended iron loading, increase of total iron, increase of free iron, extensive oxidative stress with membrane phosphatidylserine (PS) exposure in the peripheral erythrocytes, which (3) activates splenic macrophages and leads to premature destruction of the erythrocytes. Full size image We report here molecular mechanisms of mtDNA mutagenesis-associated anaemia. We show that mtDNA mutagenesis affects mitochondrial removal during erythroid development indicating that signals intrinsic to mitochondria contribute to red blood cell maturation. The consequence of mtDNA mutagenesis is respiratory chain enzymes carrying random single amino acid changes, resulting in subtle increase of ROS [9] , [33] . We show that ROS/redox signalling in erythroid maturation affects transferrin-mediated iron loading that in turn leads to an increase of total and NPBI in the peripheral blood of these animals. The presence of free iron in oxygen-carrying red blood cells is exceptionally deleterious, leading to a vicious cascade of oxidative damage and modified membrane lipid structure—even after mitochondria were successfully excluded. We show that newly synthesized red blood cells in the progeroid Mutator-mouse model carry a membrane signature of premature aging that leads to premature splenic capture and shortened lifespan of the erythrocytes. This process results in iron accumulation in the spleen with simultaneous iron deficiency in the bone marrow, despite normal nutritional iron intake. This evidence suggests that mtDNA mutagenesis induces cell-intrinsic aberration to mitochondrial removal and a major iron metabolic defect, within erythroid progenitors as well as in bone marrow and spleen. The mechanisms we have identified may be relevant to the manifestation of anemias in human mitochondrial disorders as well as those of old age where the decline in mitochondrial function and increased mtDNA mutagenesis are well documented. We show here that mitochondria regulate their own removal from maturing reticulocytes. Delayed mitochondrial clearance has been found in mouse models that are missing specific components of mitochondrial clearance pathway, including Nix [19] , [20] , Ulk1 (ref. 17 ) and Atg7 ( [34] , [35] ). Reticulocyte culture from those knock-out animals mimicked closely the mitochondrial exclusion defect we observed in the Mutators [15] , [17] , [20] . Furthermore, pharmacological inhibition of 15-lipoxygenase (15-LOX), an enzyme involved in degradation of mitochondria during reticulocyte maturation, led to an accumulation of mitochondria in a subset of mature erythrocytes [13] , [36] . Nonetheless, in all of these murine models the majority of the mature erythrocytes lacked mitochondria, suggesting considerable functional redundancy in organelle clearance during erythroid development. The Mutator mouse—a model affecting primarily mtDNA quality and not directly mitophagy-associated proteins—indicates that mitochondrial-originating signals can modify organellar exclusion. We found that the mitochondrial exclusion delay in Mutator in vitro reticulocytes was accompanied by a delay in mitochondrial depolarization, which was rescued by NAC, indicating that ROS/redox status participates in loss of membrane potential in erythroid maturation. In reticulocytes, depolarized mitochondria most often reside within autophagosomes, but depolarization is not thought to be required for mitophagy [35] . We did not find direct evidence for NAC-induced autophagy or lysosomal biogenesis, to explain NAC-enhanced mitochondrial uncoupling. This suggests that mitochondrial depolarization was not a direct consequence of mitophagy, and that mtDNA mutagenesis associated with decreased capacity to mitophagy, agreeing with a previous report [37] . In non-erythroid cells, mitophagy has been induced by chemical uncoupling of mitochondria, by mechanisms involving Pink1–Parkin-mediated pathway and Ulk1 (refs 38 , 39 , 40 ). Whether similar mechanisms regulate mitophagy during erythrocyte maturation remains to be explored. We show that the prolonged presence of mitochondria in erythrocytes is accompanied by severe aberration of iron metabolism, delayed TfR clustering and exclusion, suggesting that mitochondrial-derived signals contribute to these mechanisms. The remarkable increase of both total and free iron, inside erythrocytes and in plasma, strongly supported extended iron loading, leading to extensive oxidative stress and damage of erythrocyte membranes in Mutators. Consistently, oxidative membrane aging-markers in the newly formed red blood cells were increased, indicating premature aging of Mutator erythrocytes. Similar findings of increased oxidative stress and enhanced erythrocyte destruction have been reported in disorders of iron metabolism, as well as in sickle cell anaemia [41] , [42] . Mutator mice were originally not found to have oxidative damage in their postmitotic tissues [7] , [43] , but recent reports indicated some increase of damage [44] , as well as age-dependent increase of hydrogen peroxide [33] . In SSCs of Mutators, subtle increase of ROS has been shown to modify signalling and cause SSC dysfunction [9] . Our results show that even in an organism with wide-spread mtDNA mutagenesis in all tissues, ROS signalling and oxidative stress can affect function of a very specific cell type. In the Mutator, the iron-mediated oxidative radicals and damage have deleterious effects to red blood cell maturation, limiting the lifespan of the animals. We propose here a pathomechanistic model for mtDNA mutagenesis-linked anaemia ( Fig. 5c ). As both mitochondria and TfR-mediated iron loading are simultaneously required for haeme synthesis, and the removal of both mitochondria and TfR are tightly regulated in erythroid cell maturation, these mechanisms are likely to be synchronized. A previous report found that ROS promoted translation of TfR thereby prolonging iron loading [45] . We propose that the continued presence of mitochondria in maturing erythroid cells is signalled to TfR through subtle ROS signalling, and is magnified by mtDNA mutagenesis. Therefore, this elevated ROS signal leads to extended TfR activity and iron loading in erythroid precursors that leads to an increase of cellular iron with free oxidized—‘rusty’—iron unable to be inserted to haeme or bind oxygen. These conclusions are supported by the fact that NAC rescued TfR exclusion in Mutator erythrocytes. NAC has also been shown to increase iron regulatory protein-2 degradation, decreasing TfR activity [46] . The accumulation of NPBI inevitably induces extensive oxidative stress through Fenton reaction and leads to membrane damage that triggers splenic macrophages to capture and destroy circulating erythrocytes. Ultimately this vicious circle depletes the organism of erythrocytes and sequesters iron away from the bone marrow compromising erythropoiesis. As the anaemia in Mutator-mouse anaemia mimicked Pearson’s syndrome in humans, we searched from large clinical centres treating mitochondrial disease patients for samples from patients with acute Pearson’s anaemia. We were able to obtain samples from one rare patient, in her acute anaemic phase as well as after recovery, and showed that her peripheral erythrocytes contained mitochondria, similar to the Mutators. The rarity, common lethality of the syndrome and transient nature of Pearson’s anaemia hampered collection of a series of samples. Our intriguing findings in a single Pearson’s patient were consistent with the mechanism we established in mice with elevated mtDNA mutations, suggesting the potential for a common pathogenesis linking mitochondrial dysfunction to anaemia. Furthermore, the decreased erythroid colony forming potential of Mutator HSCs, combined with a severe maturation delay, is also typical for HSCs extracted from aged people [47] . Anaemia is an important class of human disorders affecting over 50% of 80-year-olds in the population [48] , but only 30% of aging-related anaemia can be explained by iron deficiency [49] . Since mtDNA mutations accumulate in normal aging humans [50] this raises the question whether aging-related anaemia in human population might also have mitochondrial contribution. Our findings from a progeroid mouse model anaemia suggest that related ‘rusty-when-old’ mechanisms could be important for pathogenesis of anaemia of old age. Mouse models All animal experimentation was approved by the Ethical Review Board of Finland. Mutator mice with a knock-in inactivating mutation (D257A) in the exonuclease domain of DNA polymerase gamma were used [7] . The strain was maintained by crossings with D257A/wt males and wt/wt (B57BL/6JRcc) females to prevent transmission of mtDNA mutations to germline. Experimental groups were produced by crossings with F1 generation D257A/wt females and D257A/wt males. The patient is the first child of unrelated parents. She was born after normal pregnancy, delivery and first months of life. At the age of 8 months, after respiratory infection, she developed severe anaemia with hypocellular bone marrow. A single heteroplasmic mtDNA deletion of 6 kb in size was found, the mutant mtDNA comprising about 70% of all mtDNA in peripheral blood cells. The patient was dependent on erythrocyte transfusions until the age of 20 months. By the age of 2 years, she had spontaneously recovered from the anaemia. Blood samples were taken during the acute anaemia, 2 months after previous transfusion, and a follow-up sample 15 months after the last transfusion. The control subject was an age-matched patient with medium-chain acyl-coenzyme-A dehydrogenase deficiency, a mitochondrial disease without anaemia. Informed consent was obtained from the parents of the patient and control. Terminal blood samples Mice were killed and blood was collected into EDTA tube (Greiner bio-one) by heart puncture. In the iron and 4-HNE-PA analysis, Li-heparin tubes were used, and samples from —three to five animals were pooled together to have enough sample for the analysis. Plasma and cells were separated by centrifugation and plasma was used for NPBI and 4-HNE-PA analysis (see below). Buffy coat was removed by aspiration and erythrocytes were washed twice with 0.9% NaCl. Half of packed red blood cells (RBCs) were used for NPBI analysis, and RBC ghosts were made from the remaining packed cells (see below). Blood count Blood count was performed from whole blood samples during the same day using Advia 2120i analyzer (Siemens). Assessment of maturity of the reticulocytes Intensity of ribosomal RNA staining (thiazole orange, sc-215967, Santa Cruz) was used to stage reticulocytes as immature (most intense thiazole orange (TO) signal), intermediate and mature according to standard protocol [51] . Fluorescent signal was detected by Accuri flow cytometer (Becton Dickinson) and 30,000 cells per sample were analyzed. Male mice were analyzed at the age of 6 and 11 months. Morphological analysis of erythrocytes by electron microscopy Lymphocytes and erythrocytes were separated from EDTA blood using Ficoll-Paque Plus (GE Healthcare) according to manufacturer’s instructions. Cells were fixed with 5% glutaraldehyde. Plastic embedding and sectioning were performed in the Electron Microscopy Unit in Institute of Biotechnology (University of Helsinki, Finland). Samples were analyzed using Jeol 1200 EX II transmission electron microscope. Male mice were analyzed at the age of 8 months. Induction of reticulocytosis Mice were phlebotomized to ensure sufficient amount of reticulocytes for the experiments. Two-month old mice, both females and males, were phlebotomized and 200–250 μl of blood was collected in 4 consecutive days from vena saphena. An equal volume of sterile 0.9% NaCl was given intraperitoneally, as volume replacement after each phlebotomy. Haemoglobin was monitored daily to monitor the anaemia level. On the fifth day, the mice were killed and blood was collected into EDTA tube by heart puncture. Reticulocyte culture Reticulocytes from EDTA blood were cultured as previously reported [52] . In short, EDTA blood was diluted 1:500 in reticulocyte medium, plated unto low attachment plates and maintained in a cell culture incubator with 5% CO 2, at 37 °C for 4 days. Reticulocyte medium included 30% FBS, 0.001% monothioglycerol (sc-213414, Santa Cruz), 1% deionized bovine serum albumin, 2 mM glutamine, 100 U penicillin and 0.1 mg ml −1 streptomycin in Iscove’s Modified Dulbecco’s Medium (21980-032, Gibco). Cell culture grade reagents were obtained from Sigma-Aldrich, if not otherwise noted. N-acetyl-L-cysteine treatment About 100 mg kg −1 of NAC (A7250, Sigma-Aldrich) was administered intraperitoneally after each phlebotomy, and 100 nM NAC was added to the reticulocyte culture medium. In long-term NAC treatment, study mice were given 1 mg ml −1 of N -acetyl- L -cysteine in drinking water during pregnancy, lactation and continued for the pups after weaning throughout their life. Only male mice were included in the long-term treatment and follow-up. Analysis of mitochondrial clearance in reticulocytes Cultured reticulocytes were analyzed as previously described [52] . In short, Accuri flow cytometer, nucleic acid dye TO and MitoTracker Red (Molecular Probes) were used and 30,000 cells per sample were analyzed. Cells were incubated in reticulocyte medium with 200 nM MitoTracker at 37 °C for 20 min, washed with PBS and suspended in PBS with 2 μg ml −1 thiazole orange and incubated for 40 min, followed by two PBS washes. Lasers and filters used for TO and MitoTracker Red detection were 488-nm laser with 533/30-nm filter and 640-nm laser with 675/25-nm filter. Cells were also stained with 500 nM MitoTracker Green, 1 μM TMRM (Molecular Probes), 60 nM LysoTracker Red, anti-CD71 PE (553267, Beckton Dickinson, 1 μg per 1 × 10 6 cells) and anti-Ter119 FITC (11–5921–82, eBioscience, 1 μg per 1 × 10 6 cells) and visualized using confocal microscope (Zeiss). Total iron analysis Serum/plasma total iron was analyzed using standard ferrozine method, but without deproteinization. In short, serum/plasma was diluted with 100 mM acetate buffer to reduce Fe(III) molecules to Fe(II) molecules, which makes iron soluble. Ferrozine was added to final concentration of 62.5 μM and coloured complex formed by Fe(II) and ferrozine was measured by spectrophotometer at wavelength 570 nm. Transferrin analysis Serum/plasma transferrin was analyzed using Abcam’s Transferrin Mouse ELISA kit (ab157724) according to manufacturer’s instructions. Transferrin saturation (%) was calculated by following formula: 3.825 × iron (μmol l −1 ) per transferrin (g l −1 ). Plasma and intra-erythrocyte NPBI analysis Plasma was diluted vol/vol in distilled water and desferrioxamine (DFO, D9533, Sigma-Aldrich) was added (25 μM), followed by a 30-min incubation period at −80 °C. After thawing at room temperature, samples were ultrafiltered at 3,400 g for 30 min using centrifugal filters with 30 kDa cut-off (Vivaspin 4, Sartorius Stedim Biotech GmbH). Ultrafiltrate was stored at −80 °C until analysis. The DFO excess was removed by silica (silicagel; 25–40 μm) column chromatography. The DFO–iron complex was determined by HPLC, as previously reported [24] . In short, the flow rate was 1.5 ml min −1 and the pressure stabilized to 115–125 bars. Detection wavelength was 229 nm. Packed erythrocytes were resuspended (vol/vol) in Ringer solution (125 mM NaCl, 5 mM KCl, 1 mM MgSO 4 , 32 mM HEPES, 5 mM glucose, 1 mM CaCl 2 ) pH 7.4 and erythrocyte suspension was further diluted (vol/vol) with distilled water, followed by addition of DFO and further treated similar to plasma samples. Preparation of erythrocyte membranes (RBC ghosts) Packed erythrocytes were lysed using buffer containing 5 mM KH 2 PO 4 and 0.78 mM EDTA in pH 8.0 by repeated resuspensions and centrifugations, resulting in pearly white membrane fraction. Samples were stored at −80 °C until analysis. Western blot for 4-HNE protein adducts About 30 μg of protein (RBC ghosts and plasma) were resolved on 10% SDS–PAGE gels and transferred onto a Hybond ECL nitrocellulose membrane (Bio-Rad Laboratories). After blocking with 3% non-fat milk, the membranes were incubated overnight at +4 °C with goat polyclonal anti 4-HNE antibody (1:3,000, AB5605, Millipore). After TBST washes, the membranes were incubated with secondary antibody (1:10,000, rabbit anti-goat horseradish peroxidase conjugated, Sigma-Aldrich) and detected using enhanced chemiluminescence reagents according to manufacturer’s instructions. Quantification of the bands was performed using ImageJ software. See Supplementary Fig. 4b,c for all the original blots. Analysis of PS exposure in erythrocytes Packed erythrocytes were diluted 1:250 in Ringer solution and incubated with anti-Annexin V-FITC (fluorescein isothiocyanate) in binding buffer (BD Pharmingen) according to manufacturer’s instructions. Spleen cells were first stained with anti-Ter119–PE (phycoerythrin) (1 μg per 1 × 10 6 cells), followed with Annexin V antibody (556420, Sigma-Aldrich). Fluorescent signal was detected by Accuri flow cytometer and 30,000 cells per sample were analyzed. Erythrocyte lifespan analysis Survival of erythrocytes in vivo was determined using in vivo biotinylation of erythrocytes and analysis of lifespan of the biotinylated population by FACS analysis, exactly as described in ref. 53 . In short, mice were injected intravenously with 1 mg of biotin (biotin-X-NHS, Merck Millipore) for 3 consecutive days, and 0.6 mg of biotin on the 8th day. Peripheral blood samples were collected once a week for 3 weeks and stained with streptavidin–PE (554061, BD Biosciences, 1 μg per 1 × 10 6 cells). Flow cytometric analysis Peripheral blood erythrocytes, reticulocytes and spleen were analyzed by flow cytometry. Conjugated antibodies against CD71 (TfR), Ter119, CD45 (553081, BD Biosciences), CD47 (11-0471-82, e-Biosciences) and mac3 (53-1072-82, e-Biosciences) were used as 1 μg per 1 × 10 6 cells after blocking with anti-CD16/32 to prevent unspecific staining. MitoTracker Green was used to visualize mitochondria and fluorochrome-conjugated streptavidin for biotinylated erythrocytes. Samples were analyzed using Accuri flow cytometer and 30,000–100,000 cells per sample were analyzed. The results were analyzed and visualized by FlowJo data analysis software. HSC extraction from bone marrow Tibial and femoral bone marrows were collected in DMEM (D6546, Sigma-Aldrich) from 11-month-old male mice and forwarded directly to colony forming assay. Haematopoietic colony forming assay Presence of clonogenic hematopoietic progenitors in the bone marrow was analyzed by culturing hematopoietic progenitors in MethoCult (StemCell Technologies) for myelo-erythroid progenitors according to manufacturer’s instructions. Triplicates were analyzed from each sample. Preparation of histological samples Spleens from 8-month-old males and females and femoral bones from 11-month-old males were fixed in formaldehyde according to standard protocol. Bones were decalcified in 10% EDTA prior to tissue handling and paraffin embedding. Sections (3–5 μm) were cut in objective slides for staining. Perl’s Prussian Blue iron staining was used to detect iron accumulation in spleen and bone marrow. Tissue sections were deparaffinized in xylene, followed by descending ethanol series, aqua wash and 20 min of incubation in 5% potassium ferrocyanide in 10% HCl. Nuclear counterstain was performed using 0.1% nuclear fast red Kernechtrot, followed by aqua wash, ascending ethanol series, xylene and mounting. Total protein extraction from erythrocytes RIPA buffer (25 mM Tris-HCl, 150 mM NaCl, 1% NP-40, 1% sodium deoxycholate, 0.1% SDS, pH 7.5) supplemented with protease inhibitors (88665, Pierce) was used to extract total proteins from packed and washed erythrocytes. Protein amount was not quantified, since haemoglobin interferes with measurement techniques, but instead equal volume of protein lysate from every sample was loaded to the gel. Western blot analysis Protein analysis was done using SDS–PAGE method with precast 4–20% gradient gels (Bio-Rad) with semi-dry blotting to PVDF (polyvinylidene difluoride) membrane (IPVH00010, Millipore). The membrane was blocked for 1 hour with 1% milk in TBST (Tris-buffered saline and Tween 20), and primary antibodies (anti-BNIP3L/NIX 1:2,000, #2289 ProSci and anti-GAPDH 1:2,000, #2118 Cell Signaling Technology) were incubated overnight at 4 °C. Horseradish peroxidase-conjugated secondary antibody (Pierce) was incubated for 1 hour at room temperature, followed by detection using ECL reagents according to manufacturer’s instructions (#32132 Pierce). Samples were analyzed using Chemidoc (Bio-Rad) and NIX signal was normalized against GAPDH. See Supplementary Fig. 4a for all the blots. Statistical analysis Student’s t -test was used to calculate the statistical significance of the results, and two-tailed P <0.05 was considered significant. Data are represented as mean±s.d., and two-tailed P values are shown in figures as asterisks as follows: * P <0.05, ** P <0.01, *** P <0.001 and **** P <0.0001. Linear regression analysis was used to analyze statistical significance of the difference of the slopes in BFU-E maturation and erythrocyte lifespan assay. How to cite this article: Ahlqvist, K. J. et al. MtDNA mutagenesis impairs elimination of mitochondria during erythroid maturation leading to enhanced erythrocyte destruction. Nat. Commun. 6:6494 doi: 10.1038/ncomms7494 (2015).